Sequential then interactive processing of letters and words in the left fusiform gyrus Despite decades of cognitive, neuropsychological and neuroimaging studies, it is unclear if letters are identified before word-form encoding during reading, or if letters and their combinations are encoded simultaneously and interactively. Here using functional magnetic resonance imaging, we show that a ‘letter-form’ area (responding more to consonant strings than false fonts) can be distinguished from an immediately anterior ‘visual word-form area’ in ventral occipito-temporal cortex (responding more to words than consonant strings). Letter-selective magnetoencephalographic responses begin in the letter-form area ∼ 60 ms earlier than word-selective responses in the word-form area. Local field potentials confirm the latency and location of letter-selective responses. This area shows increased high-gamma power for ∼ 400 ms, and strong phase-locking with more anterior areas supporting lexico-semantic processing. These findings suggest that during reading, visual stimuli are first encoded as letters before their combinations are encoded as words. Activity then rapidly spreads anteriorly, and the entire network is engaged in sustained integrative processing. Fluent readers distinguish between thousands of subtly different visual stimuli, associating each with a different meaning within a few hundred milliseconds. Some models of reading suppose that visual stimuli are identified as letters before their ordered combinations are identified as words, noting that brain lesions can specifically impair the ability to recognize letters [1] , or to identify single letters but not whole words [2] . Such cases are countered by studies in healthy subjects showing that letters are more quickly and accurately identified within the context of words (the ‘word superiority effect’), suggesting that letter- and word-recognition may not be sequential and separable, but rather simultaneous and integrated [3] . More recently, neuroimaging studies have identified a ‘visual word-form area’ (VWFA), showing increased hemodynamic activation to words compared with sensory controls, and centred in the left posterior fusiform gyrus (lpFg; for review see [4] , for limitations to this concept see [5] ). Critically, activation in this area to letter-strings increases with their similarity to actual words [6] , [7] , especially in more anterior VWFA [8] , suggested that it actually comprises a succession of detectors responding to progressively more abstract lexico-semantic aspects of the letter-strings. A word-selective response can also be recorded with Electroencephalography (EEG), peaking over the left occipital scalp at ∼ 140–220 ms [9] . This response has been localized to lpFg with magnetoencephalography (MEG) [10] , [11] and intracranial local field potentials (LFP) [12] , [13] , [14] . In contrast to the strong multimodal evidence for word-form processing in VWFA, the evidence for separable letter-form processing is equivocal. Although several studies have reported larger EEG responses to letter-strings as compared with false fonts (FF) over left lateral occipital scalp, it is not clear if these differ in either latency or location from word-form responses [9] , [15] . Functional magnetic resonance imaging (fMRI) provides more certain localization, but has not identified areas where letter-strings reliably evoke more activity than FF within lpFg, nor has it been able to provide information regarding the timing of these processes [8] , [16] . Here we identify a putative letter-form area immediately posterior to the VWFA with fMRI in healthy subjects, and show with MEG that letter-selective activation estimated to the putative letter-form area precedes the word-selective activation in the VWFA. Next, we use LFP recorded directly from the letter-form area using pial electrodes in epileptic patients to confirm and extend the non-invasive measures, providing converging evidence for a separate letter-form area preceding in time and anatomy of the VWFA. Finally, we show using intracranial recordings that activation of the putative letter-form area is prolonged, overlapping and phase-locked with anterior language areas during later, but not earlier, stages of reading. Letter- and word-selectivity We recorded brain activity in English readers evoked by FF arranged in a string like a word, by consonant strings (CS), and by real words (RW). We reasoned that if separate letter-form and word-form processing stages exist, they would be indexed by CS>FF, and RW>CS contrasts, respectively. Stimuli were presented every 600 ms with no gap, and the subject responded to rare (<5%) animal names. This task required the subject to attempt to read each stimulus, the cognitive process under examination. Although non-word stimuli would thus be subjected to less processing once they were identified as such, our main focus was on the first pass of neural activity occurring before definitive word identification. Hemodynamic responses First, we used fMRI in 12 healthy subjects to isolate candidate areas in lpFg. Letter-selective (CS>FF) hemodynamic activation was restricted to lpFg, and word-selective (RW>CS) processing was immediately anterior, with very little overlap ( Figs 1a and 2 ). Word-selective areas extended beyond the lpFg to traditional language areas (Wernicke’s and Broca’s), as well as cingulate gyrus and contralateral sites. In order to maximize single subject signal-to-noise-ratio (SNR) we used a block design for the fMRI modality only. Thus the subjects may have used shallower processing for the non-word stimuli, accentuating their difference from words. Furthermore, the contrast RW>CS would be expected to reveal areas processing more abstract lexical and semantic properties, as well as those processing word-forms. Nonetheless, the fMRI study accomplished its goal, to localize for further study candidate structures in lpFg that might underlie letter-form and word-form processing. 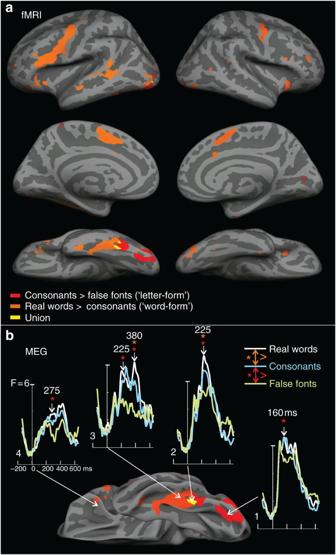Figure 1: Putative letter-form area identified with fMRI and MEG. (a)fMRI:Hemodynamic activation to letter-selective (red) and word-selective (orange) contrasts or both (yellow). (b)MEG: estimated time-courses of activation (F-values) in four regions of interest (ROI) in the left ventral occipito-temporal and orbital cortices. ROIs, centred at the ends of the arrows, were chosen based on fMRI activation. Colours (a) and asterisks (b) mark cluster-corrected differences,t-test,P<0.05;n=12 healthy subjects. MNI coordinates of the maximum activation clusters: letter-form area (−40 −78 −18), word-form area (−46 −52 −20). Figure 1: Putative letter-form area identified with fMRI and MEG. ( a ) fMRI: Hemodynamic activation to letter-selective (red) and word-selective (orange) contrasts or both (yellow). ( b ) MEG : estimated time-courses of activation ( F -values) in four regions of interest (ROI) in the left ventral occipito-temporal and orbital cortices. ROIs, centred at the ends of the arrows, were chosen based on fMRI activation. Colours ( a ) and asterisks ( b ) mark cluster-corrected differences, t -test, P <0.05; n =12 healthy subjects. MNI coordinates of the maximum activation clusters: letter-form area (−40 −78 −18), word-form area (−46 −52 −20). 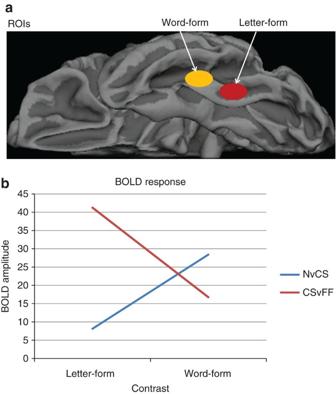Figure 2: Interaction of BOLD response to factors of task contrast and ROI. (a) Location of putative letter-form and word-form areas used for this analysis. (b) BOLD response in these areas to the letter-form contrast (CS, as compared with FF) and word-form contrast (N, novel words, as compared with CS). BOLD signal in the letter-form area (left) is very sensitive to the CS versus FF contrast but not to the N versus CS contrast, that is, it is sensitive to whether the stimulus is composed of letters but not to whether the letters compose a word. In contrast, BOLD signal in the word-form area is somewhat sensitive to whether the stimulus is composed of letters (CSvFF), but is more sensitive to whether the letters compose a word. Analysis of variance. for area (letter-form, word-form) × contrast (CSvFF, NvCS) showed a significant area × contrast interaction (P<0.05,F(11)=5.05). The BOLD response is in arbitrary units. Full size image Figure 2: Interaction of BOLD response to factors of task contrast and ROI. ( a ) Location of putative letter-form and word-form areas used for this analysis. ( b ) BOLD response in these areas to the letter-form contrast (CS, as compared with FF) and word-form contrast (N, novel words, as compared with CS). BOLD signal in the letter-form area (left) is very sensitive to the CS versus FF contrast but not to the N versus CS contrast, that is, it is sensitive to whether the stimulus is composed of letters but not to whether the letters compose a word. In contrast, BOLD signal in the word-form area is somewhat sensitive to whether the stimulus is composed of letters (CSvFF), but is more sensitive to whether the letters compose a word. Analysis of variance. for area (letter-form, word-form) × contrast (CSvFF, NvCS) showed a significant area × contrast interaction ( P <0.05, F (11)=5.05). The BOLD response is in arbitrary units. Full size image Magnetoencephalographic responses Owing to the nature of neurovascular coupling, hemodynamic measures cannot distinguish the onsets of neural processing stages that differ by less than about a second. Consequently, we turned to the millisecond accuracy of MEG to examine the time-course of processing evoked by FF, CS and RW within the regions identified by fMRI in the lpFg. By using a random stimulus order, and concentrating on first-pass processing, we were able to determine when CS>FF and RW>CS effects initially occur, before potentially confounding effects of differential processing, which could occur only after stimulus identification. MEG is mainly generated by currents within apical dendrites of cortical pyramidal cells. Currents were estimated with noise-normalized minimum norm constrained by each subject’s MRI [17] . At 160 ms, the first letter-, but not word-selective differences peak in lpFg ( Fig. 1b , area 1). Word-selective activation emerges later, peaking at 225 ms in an immediately anterior location ( Fig. 1b , area 2). At this latency, letter-selective responses are also estimated to this area. Thus, like hemodynamic activation, the earliest neural currents that were letter-selective but not word-selective were estimated to occur only in the most posterior part of lpFg. Furthermore, these letter-selective currents peaked earlier than more anterior word-selective responses. Unlike its hemodynamic response, currents in anterior fusiform gyrus showed letter-selective, as well as word-selective responses ( Fig. 1b , area 3). Dissociations between MEG and fMRI may occur because they are sensitive to different aspects of neural activity, and fMRI integrates activity over a longer time period [18] . Nonetheless, MEG confirms a succession in time and space of neural currents distinguishing first letters and then words from their respective controls, confirming the spatial succession shown by hemodynamic measures ( Fig. 3 ). 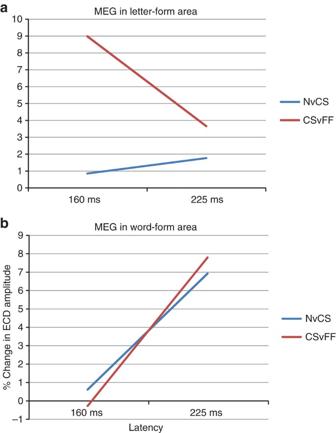Figure 3: Task contrasts across different latencies and areas. (a) Equivalent current dipole (ECD) strength in the letter-form area responds at an early latency (160 ms) to CS (CS, as compared with FF), but shows little differential response at either latency to novel words (N) versus CS. putative letter-form and word-form areas were defined by fMRI responses in the same subjects. ECD strength is estimated from MEG as the absolute difference between noise-normalized dipole strengths. (b) ECD strength in the word-form area shows little differential response to either contrast at the early latency, but responds more to words than CS, at the longer latency (225 ms). A supplementary MANOVA for area (letter-form, word-form) × latency (160, 225 ms) × contrast (CSvFF, NvCS) showed a significant area × latency interaction (P<0.05,F(1,11)=5.97). MEG responses were estimated for areas 1 and 3 as shown inFig. 1. Motivated by studies suggesting that very-early word-selective responses may be present shortly after∼100 ms50,51, we also examined MEG responses at this latency in a supplementaryt-test but failed to find any differences between conditions. Figure 3: Task contrasts across different latencies and areas. ( a ) Equivalent current dipole (ECD) strength in the letter-form area responds at an early latency (160 ms) to CS (CS, as compared with FF), but shows little differential response at either latency to novel words (N) versus CS. putative letter-form and word-form areas were defined by fMRI responses in the same subjects. ECD strength is estimated from MEG as the absolute difference between noise-normalized dipole strengths. ( b ) ECD strength in the word-form area shows little differential response to either contrast at the early latency, but responds more to words than CS, at the longer latency (225 ms). A supplementary MANOVA for area (letter-form, word-form) × latency (160, 225 ms) × contrast (CSvFF, NvCS) showed a significant area × latency interaction ( P <0.05, F (1,11)=5.97). MEG responses were estimated for areas 1 and 3 as shown in Fig. 1 . Motivated by studies suggesting that very-early word-selective responses may be present shortly after ∼ 100 ms [50] , [51] , we also examined MEG responses at this latency in a supplementary t -test but failed to find any differences between conditions. Full size image Intracranial EEG responses Although providing excellent timing, localizations of MEG generators are always subject to some uncertainty. Unambiguous localization was obtained with LFP recordings from the lpFg surface using electrodes implanted in epileptic patients for the clinical purpose of localizing seizure onset relative to eloquent cortex. Nine patients had electrodes located in the ventral occipito-temporal region of the language dominant hemisphere, and had normal verbal intelligence testing and reading ability ( Supplementary Table S1 ). Electrode contacts considered for analysis were within 1 cm of the group hemodynamic response, were distant from the ultimately determined seizure focus and from brain abnormalities identified with structural imaging, and had normal-appearing background activity with few or no epileptiform spikes or slow waves. Of 34 such contacts, 25 recorded LFP (intracranial event-related potential (ERP)) that responded during the task compared with prestimulus baseline. Of these 25 responsive contacts, 14 responded differentially to CS versus FF before 300 ms ( Fig. 4 ). As the LFP records essentially the same signal locally that the MEG records at a distance, the LFP responses directly confirm the inferred localization of MEG generators ( Supplementary Fig. S1 ). 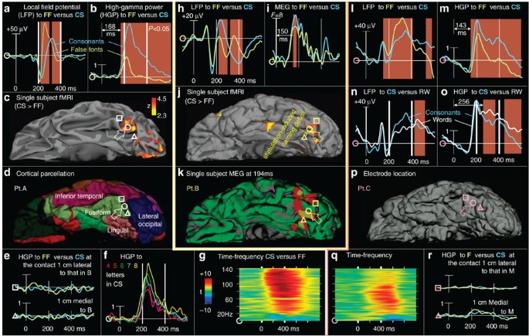Figure 4: Direct intracranial recordings confirm inferences from non-invasive fMRI and MEG. (a) Intracranial LFP (a) and HGP (b) differentiate between CS versus FF, in an electrode contact (bold white circle, open arrow) centred on fMRI activation to the same contrast in the same patient (c), at the posterior limit of the left fusiform gyrus (d). No HGP response to either CS or FF were recorded by adjacent contacts (e; responses are plotted at the same scale as inb; these adjacent contacts, which are lateral (L) or medial (M) to that inb, are marked incandd). The HGP response was highly correlated with the number of letters (f), and extended to >140 Hz (g).a,b,f, andgdisplay different recordings from the same contact. (b) Differential LFP (h) response to CS versus FF in another patient, again recorded over the left posterior fusiform cortex in a location, which showed BOLD activation (j) in the same contrast in the same patient. Electrical stimulation between this contact and the medially adjacent contact (j) disrupted naming performance. This patient also performed MEG with activation (F-values) estimated to the same area at the latency of the LFP response (i,k). (c) Differential LFP (l) and HGP (m) responses to CS versus FF over left posterior fusiform cortex (p). Although the same location responds to words versus consonants (n,o), the differential response begins >80 ms later. Again, the HGP response extends across all recorded gamma frequencies (q), and no significant response is observed in adjacent contacts (r; same scale asm). The polarity and morphology of the LFP responses (a,h,l) are highly variable as is typically seen in the vicinity of the LFP generator, presumably reflecting the exact spatial relationship of the electrode to the generator, as well as individual differences. Brown rectangles behind waveforms indicate significant condition differences using resampling statistics across individual trials. HGP is in arbitrary units. Figure 4: Direct intracranial recordings confirm inferences from non-invasive fMRI and MEG. ( a ) Intracranial LFP ( a ) and HGP ( b ) differentiate between CS versus FF, in an electrode contact (bold white circle, open arrow) centred on fMRI activation to the same contrast in the same patient ( c ), at the posterior limit of the left fusiform gyrus ( d ). No HGP response to either CS or FF were recorded by adjacent contacts ( e ; responses are plotted at the same scale as in b ; these adjacent contacts, which are lateral (L) or medial (M) to that in b , are marked in c and d ). The HGP response was highly correlated with the number of letters ( f ), and extended to >140 Hz ( g ). a , b , f , and g display different recordings from the same contact. ( b ) Differential LFP ( h ) response to CS versus FF in another patient, again recorded over the left posterior fusiform cortex in a location, which showed BOLD activation ( j ) in the same contrast in the same patient. Electrical stimulation between this contact and the medially adjacent contact ( j ) disrupted naming performance. This patient also performed MEG with activation ( F -values) estimated to the same area at the latency of the LFP response ( i , k ). ( c ) Differential LFP ( l ) and HGP ( m ) responses to CS versus FF over left posterior fusiform cortex ( p ). Although the same location responds to words versus consonants ( n , o ), the differential response begins >80 ms later. Again, the HGP response extends across all recorded gamma frequencies ( q ), and no significant response is observed in adjacent contacts ( r ; same scale as m ). The polarity and morphology of the LFP responses ( a , h , l ) are highly variable as is typically seen in the vicinity of the LFP generator, presumably reflecting the exact spatial relationship of the electrode to the generator, as well as individual differences. Brown rectangles behind waveforms indicate significant condition differences using resampling statistics across individual trials. HGP is in arbitrary units. Full size image High-gamma band power The polarity of MEG or LFP does not reliably indicate if the underlying population is producing increased or decreased neuronal activity. Such information can be derived from broadband high-gamma power (HGP), which arises from summated fast post-synaptic membrane currents and action potentials. The nine patients were implanted with a total of 1,351 electrodes of which 107 (7.9%) contacts exhibited significant task-related HGP. Of these 107, 7 (6.5%) contacts recorded greater activation to CS than FF before 250 ms, of which 6 (85%) were in lpFg, thus providing additional evidence that letter-selective activation is mainly localized to this area. Common response patterns across brain-imaging modalities The locations and timing of the LFP and HGP responses to words, CS and FF directly recorded from lpFg in patients thus showed a good correspondence to the fMRI and MEG contrasts recorded from healthy controls. In addition, excellent correspondence was observed in one patient studied with fMRI before electrode implantation ( Fig. 4a ), and in another patient studied with both fMRI and MEG recordings ( Fig. 4b ). The recording electrode on the cortical location showing CS>FF hemodynamic activation also recorded focal CS>FF LFP and HGP. The HGP response significantly differentiates between CS and FF beginning at ∼ 140–170 ms, very close to that observed with MEG in the same subject. The LFP and HGP responses were in most cases highly focal, being absent in the adjacent contacts separated by 6 mm ( Fig. 4e ). Number of letters Previous studies have found that the number of letters does not affect hemodynamic activation of the VWFA, but does affect the immediately posterior region [19] , [20] . We also found that the letter-selective HGP responses increased linearly with the number of letters ( Fig. 4f ). Specifically, in the two subjects with the highest SNR recordings, the average HGP from 200–300 ms correlated with number of letters in CS (Pearson’s r =0.96, 0.95; both P <0.01) and words (Pearson’s r =0.94, 0.88; both P <0.05) but not FF ( r =−0.32, 0.64; both P >0.2; please see Supplementary Materials for details). Thus, this correlation with number of letters does not reflect greater sensory stimulation (as it was not seen with increasing numbers of FF stimuli), and is independent of word frequency or meaning (as CS have neither). When considering the words only, there is no significant correlation with word frequency if the effects of word length are removed ( Supplementary Materials ), unlike what has been reported for the VWFA [21] . These findings show that the processing devoted by the letter-selective area to a stimulus is proportional to the number of letters it contains but is not sensitive to basic lexical properties such as frequency. These characteristics are consistent with its putative role in processing individual letters instead of whole words, and distinguish it from the VWFA. Temporal dynamics of HGP As HGP is highly correlated with hemodynamic activation [22] , the HGP responses recorded at the location of hemodynamic responses should indicate the time-course of the neural activity underlying the hemodynamic activations. In the highest SNR HGP recordings, letter-selective activity began at ∼ 150 ms after CS onset, peaked at ∼ 200 ms and continued for over 400 ms ( Fig. 4b ). Thus, although activation of the putative letter-form area begins before more anterior language areas, it is prolonged and overlaps with word-form, lexical and lexico-semantic processing. Temporal dynamics of communication between brain regions In order to obtain additional evidence regarding whether these coactivated areas are communicating, the phase-locking value (PLV) was calculated between active sites [23] . PLV measures the consistency of the relative phase of LFPs in two locations. High PLV indicates consistent synchronization of the synaptic currents in pyramidal apical dendrites between the cortical locations underlying the intracranial sensors. Such inferences are weakened in EEG or MEG by the fact that any two sensors will often record activity from the same cortical location, resulting in spurious correlations [24] . Intracranial LFP are focally sensitive to the underlying cortex and thus are not prone to this confound. PLV was strongly elevated during word processing from ∼ 170–400 ms between the lpFg sites showing letter-selectivity and other locations responding to words ( Fig. 5 ). In order to test the generality of this finding, a single-trial estimate of the PLV (PLVi) was calculated for 24 electrode-pairs, each between an lpFg electrode with early CS>FF HGP activation, and another location with temporally overlapping statistically significant differential HGP responses in the same task. Fourteen (58%) showed significantly increased PLVi (8–35 Hz; 140–300 ms) to words as compared with FF ( P <0.01; please see Supplementary Materials for details). Although the PLV indicated very-high levels of phase synchrony during the critical period while reading words, it was at chance levels before word onset, or in response to FF ( Fig. 5 ). Resting-state fMRI correlations have been reported between the VWFA and other language-related regions [25] , but other studies have given apparently contradictory results [26] . In any case, the phase-locking reported here is transient and restricted to reading, and occurs at an about one thousand times higher frequency (8–35 Hz for PLV as compared with 01–1 Hz for resting-state fMRI correlations), rendering direct comparisons problematic. The high PLV between the putative letter-form area and anterior language-related areas suggests that although early processing of the visual word during reading is sequential and modular, later processing is simultaneous and interactive across a widespread network of structures with complementary specializations. Participation by letter-selective regions in the broader language network is also implied by the picture naming deficits induced by electrical stimulation of the contacts recording letter-selective responses in one subject ( Fig. 4j ). 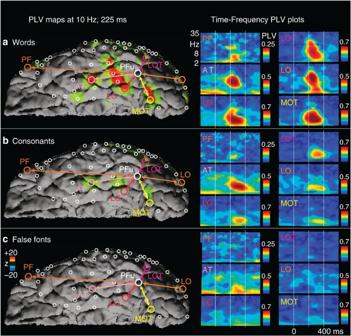Figure 5: Phase-locking values between coactivated structures suggests sustained interactions. PLV between the posterior fusiform letter-selective area (large white circle) and other simultaneously active sites (coloured circles) is increased from 160-400 ms for words (a), and consonants (b), but not for FF (c). Columns 2 and 3: Time-frequency plots of PLV between the posterior fusiform and the prefrontal (PF), anterior temporal (AT), lingual (LG), lateral occipital-temporal (LOT), lateral occipital (LO), and medial occipito-temporal (MOT) contacts. The colour bar ranges vary for a given contact-pair but are constant for a given contact-pair across all conditions. Column 1: PLV between the posterior fusiform letter-selective site and all other sites mapped onto the reconstructed brain surface at 10 Hz, at 225 ms. Colour values indicate the z-score relative to prestimulus baseline, thresholded at z>4.5. Columns 2 and 3 display the absolute size of the PLV. Figure 5: Phase-locking values between coactivated structures suggests sustained interactions. PLV between the posterior fusiform letter-selective area (large white circle) and other simultaneously active sites (coloured circles) is increased from 160-400 ms for words ( a ), and consonants ( b ), but not for FF ( c ). Columns 2 and 3: Time-frequency plots of PLV between the posterior fusiform and the prefrontal (PF), anterior temporal (AT), lingual (LG), lateral occipital-temporal (LOT), lateral occipital (LO), and medial occipito-temporal (MOT) contacts. The colour bar ranges vary for a given contact-pair but are constant for a given contact-pair across all conditions. Column 1: PLV between the posterior fusiform letter-selective site and all other sites mapped onto the reconstructed brain surface at 10 Hz, at 225 ms. Colour values indicate the z-score relative to prestimulus baseline, thresholded at z>4.5. Columns 2 and 3 display the absolute size of the PLV. Full size image This study replicated previous studies showing word-selective hemodynamic activation in lpFg [4] , and then demonstrated letter-selective activation in the posteriorly adjacent area. Previous studies recording the hemodynamic response to CS and FF have either not directly compared them [27] , not reported their comparison [28] , found no differences in the lpFg [16] or found only locations with FF>CS [8] . In most cases, these studies used low-level tasks in order to prevent the possible confound of differential stimulus processing, but this may have unintentionally biased them against specific letter- or word-form processing. We used a high-level task that required reading for meaning and were able to avoid the possible confound by concentrating on first-pass processing probed with high-temporal resolution electromagnetic techniques. Owing to the random stimulus order each stimulus could be a word, and thus had to be processed initially as if it were a word. Eventually, FF were identified as such, attenuating further lexico-semantic processing. However, identification of the stimulus as FF must have occurred after the stage of interest because the stage of interest is exactly that which performs such identification. Owing to the high-temporal resolution of MEG and electrocorticography (ECoG), we observed the activity of each stage without contamination by other stages, and distinguished which anatomical location selectively responded to CS versus FF at the shortest latency, even though many structures eventually showed such effects due to both feedforward and feedback influences at longer latencies. It is possible that FF could have been determined very rapidly to not be letters and this resulted in fewer resources being devoted to their further processing. Similarly, CS may have been rapidly determined to have no vowels, and thus evoked shallower processing than RW. If so, it is possible that our measure of CS processing (CS minus FF) was incomplete, for example, in that not all letters were identified during this shallow processing. However, we note that our task, which requires reading for meaning, is more likely to encourage letter identification than the perceptual tasks, which strive for identical processing of FF, CS and RW. Indeed, activation by CS of the putative letter-form area was proportional to the number of letters in the string, suggesting that all letters were processed. Finally, even if the letters in CS were not completely processed in our task (that is, as much as letters in RW), the result would be to decrease the effect size that we observed, not change their interpretation. Several studies have compared responses with letters versus symbols, sometimes finding greater fMRI activation in lpFg with consistent EEG responses [29] . Using a low-level task, Vartiainen et al. [30] did not detect greater fMRI activation to words or letters than to symbols, and other controls in lpFg, but were able to fit dipoles with greater activity to letters in lateral temporo-occipital cortex. Other studies have found that this area may show fMRI activation with attention [31] or working memory [32] for single letters as compared with symbols. Differential MEG activity to symbols has also been localized at early latencies to more postero-medial occipital areas [10] . This may correspond to the most posterior lpFg differential fMRI activation noted in the current study ( Fig. 1b ). A previous intracranial study failed to find any difference in HGP or LFP evoked by FF compared with CS [14] . However, this study also used a perceptual task, and sampled the sulci surrounding lpFg with depth electrodes. We recorded from the ventral surface of the lpFg, where the responses were highly focal. Additional studies are needed to determine if the letter-form area requires a reading task for full activation, and if it extends anatomically from the crown of the lpFg into the surrounding sulci. Additional studies are also needed to determine if this area responds to stimuli besides letters and words. Using the excellent temporal resolution of MEG we found that the letter-selective activation in lpFg precedes the more anterior word-selective activity. We confirmed the timing and anatomical location of the letter-form responses identified with the non-invasive measures with direct intracranial recordings of LFP and HG, and further demonstrated that these responses comprise increased synaptic processing. Our finding that letter-form and word-form processing are arranged sequentially in the lpFg is consistent with previous studies of reading showing relatively greater activation to higher order lexical and ultimately semantic stimulus properties in more anterior locations in humans with fMRI [8] , [33] , and MEG [34] , [35] . Intracranial recordings confirm that the first sweep of activation along the ventral stream extends to Broca’s region [14] , [36] , and comprises a current sink in layer IV with sharply increased firing [37] . In the anteroventral temporal lobe, first-pass activity to words may even be selective for the semantic category of the word [38] . These findings are also consistent with the general posterior-to-anterior gradient in the complexity of visual stimulus processing in the ventral stream demonstrated with single-unit recordings in monkeys [39] . Neural activity in the putative letter-form area remained strongly elevated during reading for hundreds of millseconds following the initial letter-selective activation. This later processing could be sensitive to multiple constraints, and preceded the behavioural response. Furthermore, during these later stages, widely distributed areas were activated to words, and their activity became strongly but transiently phase-locked with the lpFg electrodes showing early letter-form responses, especially when reading words. These results resemble the transient phase-locking that occurs between the fusiform face area and more anterior sites in the right hemisphere [40] , adding to the many parallels, which have been found between face and word recognition [4] , [41] , [42] . Thus, following the initial feedforward sweep, the current HGP and PLV results strongly support a sustained and interactive co-activation of a network of sites contributing to reading. This could provide the substrate for distributed calculation of word identity and meaning [5] , an interpretation that is supported by the disruption of naming by stimulation of the putative letter-form area in one patient. The top–down influences may also underlie the word superiority effect [3] . Alternatively, it is possible that lpFg stimulation disrupted naming by interfering with remote processing, and that top–down information to the putative letter-form area serves only as a training signal to help refine processing that is essentially sensory pattern recognition. In either case, our results suggest that words are processed first sequentially in stages with increasing complexity [4] , and then in parallel in multiple areas encoding complementary properties [43] . Participants Twelve healthy right-handed subjects underwent fMRI testing, and a separate group of 12 healthy subjects underwent MEG testing. In addition, we analysed LFP from nine patients implanted with intracranial electrodes while performing the task ( Supplementary Table 1 for patient characteristics). Electrodes were implanted to localize seizure onset before contemplated surgical treatment. One of these patients was also studied with fMRI during the same task before surgery, and another with both fMRI and MEG. Subjects gave written informed consent to participate in this study, and the study was approved by the New York University Medical Center (NYUMC) and University of Californa's Instituional Review Boards (UCSD IRBs) in accordance with the Declaration of Helsinki. Semantic judgment task Stimuli were white letters on a black background in Arial font at 4° visual angle, comprising RW, previously presented ‘old’ words (OW), non-pronounceable consonant letter-strings (CS), FF stimuli and 40 target words. FF were alphabet-like characters that matched a real letter in the English alphabet in size, number of strokes, total line length and curvature ( Table 1 ). FF strings were each matched to a RW in the number of characters. Subjects pressed a button in response to low-frequency target words representing animals. RW were 4–8 letter nouns, with a written lexical frequency of 3–80 per 10 million [44] . Tasks were programmed using Presentation software (Neurobehavioural Systems, Inc). Table 1 Stimuli used for semantic judgment tasks. Full size table The same design was used for both MEG and iEEG. We presented 400 each RW, OW, CS and FF, plus 80 targets pseudo-randomly with the constraint that each condition was preceded by every other condition with equal likelihood. Stimulus exposure and stimulus onset asynchrony were both 600 ms. Throughout the experiment, each CS and FF stimulus was only presented once. Here we report results on the RW, CS and FF comparisons; later responses to stimulus repetition are reported elsewhere [45] . Subjects detected 83% (s.d.=12.2) of the targets in the MEG task with a mean reaction time of 694 ms (s.d.=92 ms). They detected 78% (s.d.=13.8) during iEEG recordings (chance=4.8%) with a mean reaction time of 744 ms (s.d.=121 ms). As the reaction time (RT) often exceeded the stimulus onsetasynchrony (SOA), the trials following targets were excluded from averages. A blocked version of the semantic judgment task was designed for fMRI in order to maximize SNR, with 30 blocks including 5 blocks each of RW, OW and CS, and 15 blocks of FF. Each block contained 40 words of one stimulus type, plus two targets. Blocks of RW and CS were presented in random order. Subjects detected 84% (s.d.=9.2) of the targets. Mean reaction time was 688 ms (s.d.=76 ms). MRI analysis Twelve healthy subjects (six males, mean age: 23, range 19–36) underwent fMRI testing. Each subject was right-handed and free of neurological impairments. Handedness was assessed with the Edinburgh Handedness Inventory [46] . The 3T MRI data were acquired and analysed using FreeSurfer, FSL, and custom software as previously described [45] . Letter-specific activation was defined as increased BOLD to CS versus FF, as they were closely matched on basic visual features. Similarly, word-specific activity was defined as increased BOLD to RW versus CS. Larger responses to FF are common, with EEG, as well as BOLD, especially in the right hemisphere [9] , [15] . As such responses are thought to reflect the novelty of FF rather than template-matching [16] , we omitted them from our study. Functional MRI data were preprocessed using FSL ( www.fmrib.ox.ac.uk/fsl ). For each subject, motion correction was performed using FLIRT [47] , and data were spatially smoothed using a 5-mm full width half-maximum Gaussian kernel, grand-mean intensity normalized, high-pass filtered at sigma=50 sm and pre-whitened using FILM [48] . Functional scans were coregistered to T1-weighted images [47] , [49] , and analysed using FMRI Expert Analysis Tool Version 5.90, part of FSLs FMRIB’s software library. BOLD parameter estimates (beta-weights) were averaged across the two runs for each contrast of interest (RW>CS and CS>FF). Percent signal change was calculated in MATLAB (The Mathworks, Natrick, MA) by multiplying the beta-weights by 100 × the regressor height and dividing by the mean functional volume. Individually averaged functional data were then resampled from each volume to each individual’s native surface, then from native surface to spherical atlas space for surface-based group analysis. MEG analysis MEG signals were recorded from 204 planar gradiometers as previously described [11] . Distributed source estimates of cortical activity were calculated from gradiometer data using dynamic statistical parametric mapping and cortical dipole constraints derived from each individual’s reconstructed MRI [17] . Peak amplitudes from each subject in fMRI-based regions of interests were entered into analysis of variance. Intracranial EEG analysis LFP were recorded from intracranially implanted subdural electrodes (AdTech medical Instrument Corp., WI, USA) in patients undergoing elective monitoring of medically intractable seizures ( Supplementary Table S1 for patient demographics), with implant sites over the left ventral occipito-temporal cortex in nine patients. A large number of additional brain areas were sampled, including regions that were subsequently determined to be non-epileptogenic. Patients were native English speaking and left language dominant, with average performance on cognitive, language and reading tests and normal language organization as indicated by cortical stimulation mapping, when available. Only electrode contacts outside the seizure onset zone and with normal interictal activity were included in the analysis. In each case, the source of the patient’s epilepsy was thought to be focal and in an operable brain region. Electrode placement was based entirely on clinical grounds for identification of seizure foci and eloquent cortex during stimulation mapping, and included grid (8 × 8 contacts), depth (1 × 8 contacts) and strip (1 × 4 to 1 × 12 contacts) electrode arrays with 10 mm inter-electrode spacing centre-to-centre. Subdural grid and strip contacts were 4 mm in diameter; consequently the distance between contacts was 6 mm. A large number of brain areas was sampled, with coverage extending widely into regions that were subsequently determined to be non-epileptogenic. All nine patients met the following strict selection criteria: (1) left language lateralization as indicated by Wada testing; (2) cognitive and language abilities in the average range, including language and reading ability, as indicated by formal neuropsychological testing ( Supplementary Table S1 ); (3) native English speaking; (4) normal language organization as indicated by cortical stimulation mapping, when available; (5) above 75% performance on the semantic judgment task; and (6) electrode strips sampling from the left ventral occipito-temporal cortex. In addition, only electrode contacts outside the seizure onset zone and with normal interictal activity were included in the analysis. EEG activity was recorded at 400 Hz with a Nicolet 128 channel clinical amplifier (0.1 Hz–200 Hz) or at 1000 Hz with a custom-design 256 channel recording system (0.1 Hz–500 Hz). The precise localization of each electrode was computed by coregistering two T1-weighted MRIs, one obtained preoperatively and one on the day after implant surgery with the electrodes in place. A spatial optimization algorithm was used to integrate known information from the array geometry and intra-operative photos to achieve high spatial accuracy of the electrode locations in relation to the cortical MRI surface. Electrodes were visualized on the reconstructed pial surface from T1-weighted MRI scans using Freesurfer v4.1. For anatomical orientation, the Freesurfer generated cortical parcellations were overlaid onto the reconstructed surface ( Fig. 4d ). Data were analysed in Matlab using Fieldtrip and custom routines. Statistical comparison across stimulus types used a nonparametric randomization test with temporal clustering. Phase-locking value [23] , as well as a single-trial analogue ( Supplementary Methods ) were calculated between responsive subdural electrode contacts. How to cite this article: Thesen T. et al. Sequential then interactive processing of letters and words in the left fusiform gyrus. Nat. Commun. 3:1284 doi: 10.1038/ncomms2220 (2012).